Dynamic force-induced direct dissociation of protein complexes in a nuclear body in living cells Despite past progress in understanding mechanisms of cellular mechanotransduction, it is unclear whether a local surface force can directly alter nuclear functions without intermediate biochemical cascades. Here we show that a local dynamic force via integrins results in direct displacements of coilin and SMN proteins in Cajal bodies and direct dissociation of coilin-SMN associated complexes. Spontaneous movements of coilin increase more than those of SMN in the same Cajal body after dynamic force application. Fluorescence resonance energy transfer changes of coilin-SMN depend on force magnitude, an intact F-actin, cytoskeletal tension, Lamin A/C, or substrate rigidity. Other protein pairs in Cajal bodies exhibit different magnitudes of fluorescence resonance energy transfer. Dynamic cyclic force induces tiny phase lags between various protein pairs in Cajal bodies, suggesting viscoelastic interactions between them. These findings demonstrate that dynamic force-induced direct structural changes of protein complexes in Cajal bodies may represent a unique mechanism of mechanotransduction that impacts on nuclear functions involved in gene expression. It is well established that mechanical forces can influence functions of living cells, tissues and organisms. However, despite significant progress in past decades in understanding cellular mechanotransduction [1] , [2] , [3] , [4] , [5] , [6] , it is still not clear how mechanical forces applied at the cell surface alter nuclear functions of the cell. One prevailing model suggests that a local force applied at the cell surface might be able to influence the nuclear functions indirectly via induced translocation and/or diffusion of signalling molecules from the cytoplasm into the nucleus [7] . Alternatively, a local surface force, via force propagation along cytoskeletal-nuclear linkages, is speculated to directly alter nuclear functions by affecting activities of molecules inside the nucleus [3] . It has been demonstrated that a surface force/deformation via integrins can alter the gross shape of the nucleus [8] , resulting in direct deformation of nucleoli [9] , and that the nuclear lamina containing Lamin A/C is important in nuclear mechanical properties [10] , [11] , [12] , [13] . These findings suggest that it is possible that mechanical forces at the cell surface might directly alter nuclear functions via force propagation from the extracellular matrix (ECM) to the nucleus, but so far, experimental evidence is lacking. We hypothesize that a local surface force can directly alter nuclear functions via changing the protein–protein (and likely protein–RNA) associations. In this study, we provide evidence for force-induced direct dissociation of major multi-protein complex in the Cajal body (CB), a prominent nuclear body. CBs are evolutionarily conserved nuclear domains found in yeast, plant and animal cells and are critical for the biogenesis and recycling of several classes of small nuclear ribonucleoprotein (snRNP) complexes involved in pre-mRNA splicing and pre-ribosomal RNA processing [14] , [15] , and assembly and delivery of telomerase to telomeres [14] , [15] , [16] , [17] . Knockout of coilin, a marker protein of a CB, reduces viability and fertility in mice [18] and loss of SMN protein leads to spinal muscular atrophy [19] . Recent advances in our understanding of the formation, dynamics and function of CBs suggest that the CBs form as a direct reflection of activity of highly expressed genes with which they are physiologically associated [20] , [21] , [22] . Our present study demonstrates that local mechanical forces applied at the cell surface can directly alter protein–protein interactions in a nuclear body within the nucleus. A local surface force directly dissociates coilin from SMN To investigate whether a surface force applied via integrins could directly deform nuclear proteins in the CBs, we transiently co-transfected HeLa cells with two major essential CB components critical for its structural integrity, CFP-SMN and YFP-coilin [16] ( Fig. 1a ). We quantified their displacements that were synchronized with the oscillatory loading applied via an RGD-coated magnetic bead ( Fig. 1b ). We employed an established synchronous detection approach that could detect external-stress-induced nanoscale displacements at ~4 nm resolution while filtering out spontaneous movements [23] , [24] . Both CFP-SMN and YFP-coilin in the same CB were directly displaced by the external dynamic force applied on the cell surface, but SMN exhibited greater displacements in response to the same force ( Fig. 1c ), suggesting that differential displacements of coilin and SMN might lead to dissociation of the protein–protein complex, which is known to interact with each other inside the CB [25] . To further determine whether the applied surface force had any direct impact on the dissociation of the coilin from the SMN in the CB, we applied a quick instant force (a step-function) with the magnetic bead via the integrins and quantified the flourescence resonance energy transfer (FRET) changes of the CFP-SMN (the donor) and YFP-coilin (the receptor) protein pairs. The FRET ratio of CFP-SMN to YFP-coilin rapidly increased within 350 ms in response to the applied stress ( Fig. 1d ). The emission intensity of the protein pairs was anti-correlated: CFP-SMN intensity increased while YFP-coilin intensity decreased ( Fig. 1e ). This is strong evidence for a FRET change, suggesting that SMN were dissociated away from coilin by force. Varying force magnitudes revealed that the threshold stress for the FRET change was ~14–17 Pa and that the FRET change reached a plateau by ~350 ms ( Fig. 1f ). Turning off the applied force did not return the FRET ratio of CFP-SMN to YFP-coilin back to the pre-force level, suggesting that the force-induced structural changes to the protein pairs were 'plastic' or 'permanent', which lasted at least 10 s ( Fig. 1g ). To further examine the plasticity of dissociation of the protein complex, we quantified mean square displacements (MSDs) of both proteins before, during and after a cyclic stress application. Both coilin and SMN inside the same CB exhibited constrained diffusion behaviours and had almost identical spontaneous MSDs before stress application ( Fig. 1h ), suggesting that they were tightly associated and moved as a single entity. Both responded synchronously to the cyclic stress ( Fig. 1h ), suggesting that the proteins were directly displaced by the applied stress, but coilin had much greater spontaneous MSDs than SMN after stress application ( Fig. 1h ), indicating that coilin was tethered less tightly than SMN after stress application. Taken together, these data strongly suggest that an external force on the cell surface induced direct differential displacements between SMN and coilin, which resulted in the increased distances and thus the FRET change between these two proteins. 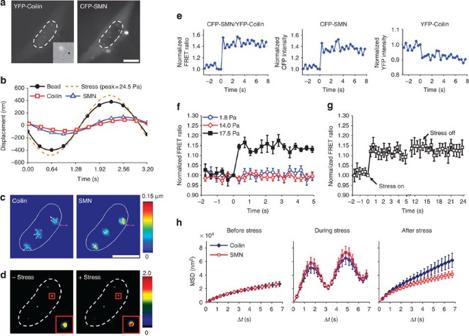Figure 1: A local surface force directly dissociates coilin from SMN in the CB in the nucleus. (a) Fluorescence images of a HeLa cell transfected with CFP-SMN and YFP-coilin (inset is the bright-field image of the cell; black dot shows the bead). Nucleus is outlined with dashed line. Scale bar, 10 μm. (b) Displacements of the magnetic bead and of the CB proteins SMN and coilin as a function of cyclic forces (0.3 Hz). Displacements of the bead, coilin and SMN were all synchronized with the applied stress (peak magnitude=24.5 Pa). (c) Displacement maps of coilin and SMN within the nucleus of the same cell. White arrows indicate direction of displacement, and the colour bar indicates the displacement magnitude. Pink arrow represents the direction of bead centre displacement (not drawn to scale). Scale bar, 10 μm (d) FRET ratio map of force-induced dissociation of coilin and SMN. Inset shows an enlarged CB with FRET changes when stress is applied. (e) A representative time course plot of CFP-SMN and YFP-coilin anti-correlation in response to force. (f) FRET ratio change between coilin and SMN by mechanical is stress-magnitude-dependent and rapid (<0.35 s). Each load was applied to a cell only once.N=5 CBs for stress of 17.5 Pa; 40 for 14 Pa; 95 for 1.8 Pa. (g) Stress-induced structural change to CB protein pairs is 'plastic'. A step load of 24.5 Pa was applied.n=13. All data points in (e), (f) and (g) were normalized to time zero when a step load was applied. (h) The dynamics of coilin and SMN were quantified before, during and after application of an oscillatory stress (24.5 Pa peak stress at 0.3 Hz). (P<0.05 when Δt>5.12 s).n=106 CBs. Mean±s.e.m.; data are pooled from >4 independent experiments for each sub-figure. A two-tailed Student'st-test was used to generatePvalues. Figure 1: A local surface force directly dissociates coilin from SMN in the CB in the nucleus. ( a ) Fluorescence images of a HeLa cell transfected with CFP-SMN and YFP-coilin (inset is the bright-field image of the cell; black dot shows the bead). Nucleus is outlined with dashed line. Scale bar, 10 μm. ( b ) Displacements of the magnetic bead and of the CB proteins SMN and coilin as a function of cyclic forces (0.3 Hz). Displacements of the bead, coilin and SMN were all synchronized with the applied stress (peak magnitude=24.5 Pa). ( c ) Displacement maps of coilin and SMN within the nucleus of the same cell. White arrows indicate direction of displacement, and the colour bar indicates the displacement magnitude. Pink arrow represents the direction of bead centre displacement (not drawn to scale). Scale bar, 10 μm ( d ) FRET ratio map of force-induced dissociation of coilin and SMN. Inset shows an enlarged CB with FRET changes when stress is applied. ( e ) A representative time course plot of CFP-SMN and YFP-coilin anti-correlation in response to force. ( f ) FRET ratio change between coilin and SMN by mechanical is stress-magnitude-dependent and rapid (<0.35 s). Each load was applied to a cell only once. N =5 CBs for stress of 17.5 Pa; 40 for 14 Pa; 95 for 1.8 Pa. ( g ) Stress-induced structural change to CB protein pairs is 'plastic'. A step load of 24.5 Pa was applied. n =13. All data points in ( e ), ( f ) and ( g ) were normalized to time zero when a step load was applied. ( h ) The dynamics of coilin and SMN were quantified before, during and after application of an oscillatory stress (24.5 Pa peak stress at 0.3 Hz). ( P <0.05 when Δ t >5.12 s). n =106 CBs. Mean±s.e.m. ; data are pooled from >4 independent experiments for each sub-figure. A two-tailed Student's t -test was used to generate P values. Full size image We next examined whether force-induced displacements of coilin or SMN in the nucleus were dependent on the distance between the site of force application and the CB. The magnitudes of SMN or coilin displacements decreased only slowly as the distance increased ( Supplementary Fig. S1 ); there were significant force-induced displacements of both proteins even when the local force (the bead) was placed >27 μm away from the CB, suggesting the force transmission pathway from the cell surface to the CB was concentrated along the force-bearing cytoskeletal-nuclear structures and that stress field did not follow the decay pattern from the homogeneous material prediction [24] . Structural basis for dissociation of coilin from SMN by force To further investigate the structural basis of stress transmission to the nucleus, we quantified changes of FRET ratio of CFP-SMN to YFP-coilin when different cytoskeletal or nuclear structural components were specifically disrupted or knocked down. Treatment with Latrunculin A, an F-actin disrupter, or blebbistatin, a myosin II inhibitor, but not colchicine, a microtubule-disrupting agent, prevented the force-induced FRET changes ( Fig. 2a ; Supplementary Fig. S2 ), suggesting that intact F-actin and myosin II, but not microtubules, are indispensable for force transmission from the cell surface to the CB in the nucleus. Knocking out Lamin A/C, a critical nuclear filament underneath the nuclear envelope, also abolished force-induced FRET changes ( Fig. 2a ), indicating the essential role of Lamin A/C in force transmission to the CB. Consistent with the necessary role of Lamin A/C in force transmission into the nucleus, using mCherry-Lamin A as a marker of the nuclear envelope, we observed deformation of the nuclear envelope in response to the local force on the cell surface ( Fig. 2b,c ; Supplementary Movie 1 ). Knocking out plectin, a linking protein connecting intermediate filaments to the nuclear envelope, did not have any effect on stress-induced FRET change ( Fig. 2a ; Supplementary Fig. S2 ), suggesting that plectin does not have an essential role in mediating force to the CB. Taken together, these results suggest that the applied stress was directly transmitted into the CB across the nuclear envelope via F-actin-LINC (linker of nucleoskeleton and cytoskeleton)-nuclear lamina structural pathways. 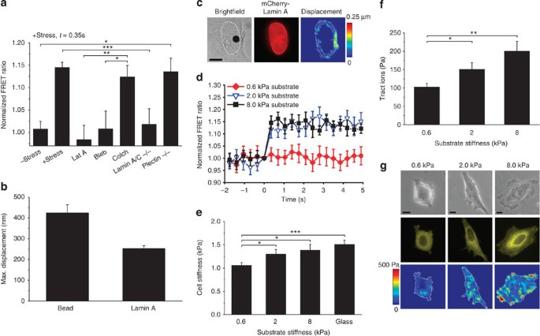Figure 2: Structural basis for force-induced dissociation of coilin from SMN. (a) Normalized FRET ratio of SMN-coilin at 0.35 s of stress application in cells treated with inhibitors or knockouts of cytoskeletal proteins or nuclear proteins. F-actin was disrupted with Latrunculin A (Lat A, 1 μM for 10 min,n=85) or myosin II was inhibited with Blebbistatin (Bleb, 50 μM for 20 min,n=58), microtubules were disrupted with colchicine (Colch, 10 μM for 15 min,n=5) (+stress; a step function of 17.5 Pa). Lamin A/C knockouts (n=43) blocked stress-induced FRET changes but Plectin knockouts (n=10) did not. (b) Stress applied at the apical surface of cell induces deformation of the nuclear envelope. Maximum displacements (Max. displacement) are plotted for the magnetic bead and for the mCherry-Lamin A-labelled nucleus in response to a cyclic stress (24.5 Pa at 0.3 Hz);n=6 cells. (c) Bright-field, fluorescent (mCherry-Lamin A), and displacement map images of a HeLa cell nucleus. Black dot on bright-field image shows the RGD-coated magnetic bead. Nucleus is outlined with white dashed lines. Scale bar, 10 μm. White arrows indicate direction of displacement, and the colour bar indicates the displacement magnitude. Pink arrow represents the direction of bead centre displacement (not drawn to scale). (d) Stress-induced dissociation of SMN-coilin in cells cultured on 8 kPa (n=10) and 2 kPa (n=8) substrates, but not on 0.6 kPa (n=55) substrate. A step load was applied at time zero, and all FRET ratios were normalized to that time point. (e) Stiffness (Young's modulus) of HeLa cells increases with the substrate stiffness. On substrate of 0.6, 2 and 8 kPa, or glass,n=77, 96, 77 or 146 cells. (f) RMS traction of the cell increases with substrate stiffness.n=9, 7 and 8 cells on substrates of 0.6, 2 and 8 kPa. (g) Phase-contrast images, corresponding YFP-actin images, and traction map images of HeLa cells cultured on 0.6, 2 and 8 kPa substrates. Scale bar, 10 μm. Mean±s.e.m. data are from at least 4 separate experiments for each sub-figure (*,P<0.05; **,P<0.01; ***,P<0.001).P-values were obtained using the two-tailed Student'st-test. Figure 2: Structural basis for force-induced dissociation of coilin from SMN. ( a ) Normalized FRET ratio of SMN-coilin at 0.35 s of stress application in cells treated with inhibitors or knockouts of cytoskeletal proteins or nuclear proteins. F-actin was disrupted with Latrunculin A (Lat A, 1 μM for 10 min, n =85) or myosin II was inhibited with Blebbistatin (Bleb, 50 μM for 20 min, n =58), microtubules were disrupted with colchicine (Colch, 10 μM for 15 min, n =5) (+stress; a step function of 17.5 Pa). Lamin A/C knockouts ( n =43) blocked stress-induced FRET changes but Plectin knockouts ( n =10) did not. ( b ) Stress applied at the apical surface of cell induces deformation of the nuclear envelope. Maximum displacements (Max. displacement) are plotted for the magnetic bead and for the mCherry-Lamin A-labelled nucleus in response to a cyclic stress (24.5 Pa at 0.3 Hz); n =6 cells. ( c ) Bright-field, fluorescent (mCherry-Lamin A), and displacement map images of a HeLa cell nucleus. Black dot on bright-field image shows the RGD-coated magnetic bead. Nucleus is outlined with white dashed lines. Scale bar, 10 μm. White arrows indicate direction of displacement, and the colour bar indicates the displacement magnitude. Pink arrow represents the direction of bead centre displacement (not drawn to scale). ( d ) Stress-induced dissociation of SMN-coilin in cells cultured on 8 kPa ( n =10) and 2 kPa ( n =8) substrates, but not on 0.6 kPa ( n =55) substrate. A step load was applied at time zero, and all FRET ratios were normalized to that time point. ( e ) Stiffness (Young's modulus) of HeLa cells increases with the substrate stiffness. On substrate of 0.6, 2 and 8 kPa, or glass, n =77, 96, 77 or 146 cells. ( f ) RMS traction of the cell increases with substrate stiffness. n =9, 7 and 8 cells on substrates of 0.6, 2 and 8 kPa. ( g ) Phase-contrast images, corresponding YFP-actin images, and traction map images of HeLa cells cultured on 0.6, 2 and 8 kPa substrates. Scale bar, 10 μm. Mean±s.e.m. data are from at least 4 separate experiments for each sub-figure (*, P <0.05; **, P <0.01; ***, P <0.001). P -values were obtained using the two-tailed Student's t -test. Full size image It is known that substrate rigidity has profound influence on cellular functions [26] . Force-induced FRET changes were observed in HeLa cells plated on 2 kPa and 8 kPa substrates, similar to those FRET changes observed in cells plated on rigid dishes, but not in cells plated on 0.6 kPa substrates ( Fig. 2d ). HeLa cells have a maximum stiffness (cell stiffness measured on a rigid dish) of ~1.51 kPa ( Fig. 2e ) and express ample actin bundles and high tractions on 2 and 8 kPa, but not on 0.6 kPa substrate ( Fig. 2f,g ). Together with the above data, this suggests that substrate rigidity regulates force-induced nuclear protein dissociation via controlling tension of the actin bundles in the cytoskeleton for long-distance force propagation. Other protein pairs exhibit different force-induced changes Next, we analysed how the local surface force affects interactions between the major interacting partners of coilin and SMN in CBs. Coilin and SMN are self-interacting proteins and their interaction is mediated by WRAP53 that is also able to self-interact [27] . Importantly, both coilin and SMN interact with spliceosomal snRNPs [28] . In addition, coilin interacts with the nucleolar chaperone Nopp140 on its amino terminus [29] and with the U4/U6 snRNP assembly factor SART3 (ref. 30 ). In the absence of external stress, spliceosomal snRNP core SmE-SmG proteins had the lowest baseline CFP/YFP emission ratios (~0.3), followed by coilin-coilin, coilin-SmE, coilin-Nopp140, WRAP53-WRAP53, coilin-WARP53, coilin-SART3, SMN-WRAP53, SMN-coilin, SMN-SMN, SMN-SmG and SMN-SART3 (~0.8) ( Fig. 3a ), suggesting that baseline distances between two proteins were closest for snRNP proteins of the Sm ring SmE-SmG and farthest for SMN-SART3 complexes. Interestingly, CFP-fibrillarin (a methylase that binds to SMN in the CB [31] ) and YFP-coilin in the CB exhibited even higher baseline emission ratios than SMN-SmG, reaching almost 1.0 ( Fig. 3a ), consistent with previously published data that fibrillarin and coilin do not directly interact with each other [14] and that they might be far apart (~>10 nm) (a negative control). After a quick step-function force was applied, coilin-coilin self-interaction exhibited greatest FRET ratio increases from baseline values, followed by coilin-SmE, WRAP53-WRAP53, coilin-Nopp140, SMN-coilin, coilin-SART3, coilin-WARP53, SMN-SMN, SMN-SmG and SMN-WRAP53 ( Fig. 3b ; Supplementary Figs S3 and S4 ). These results suggest that when these protein complexes were exposed to the same magnitudes of stress, their respective FRET ratio changes were, in general, inversely proportional to their baseline distances between the two proteins, except for SMN-coilin, which had larger FRET ratio changes than SMN-WRAP53. This suggests that distances between the SMN-coilin protein pairs increased more than predicted from their baseline values. Fibrillarin-coilin and SMN-SART3 pairs did not exhibit any FRET change from the baseline ( Fig. 3b ; Supplementary Figs S3 and S4 ), consistent with the baseline data that fibrillarin–coilin and SMN-SART3 are already too far apart at baseline, so that they are beyond the detection range of FRET changes. In contrast, SmE and SmG proteins strongly interact within the heteroheptameric ring of the spliceosomal snRNP core structure. It is likely that they could not be dissociated by the magnitude of the applied stress and, thus, did not exhibit FRET ratio change on stress ( Fig. 3b ). 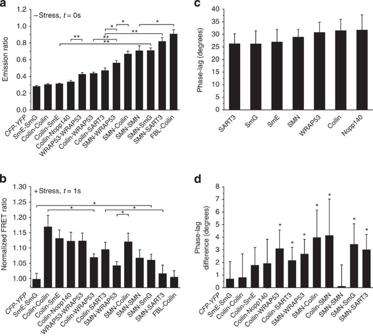Figure 3: Different protein complexes in the CB have distinct association characteristics. (a) Baseline emission ratios of SmE-SmG (n=85), coilin-coilin (n=56), coilin-SmE (n=134), coilin-Nopp140 (n=64), WRAP53-WRAP53 (n=99), coilin-WRAP53 (n=140), coilin-SART3 (n=138), SMN-WRAP53 (n=64), SMN-coilin (n=53), SMN-SMN (n=48), SMN-SmG (n=100), SMN-SART3 (n=73) and Fibrillarin (FBL)-coilin (n=32) before stress application. No significant difference was observed between coilin-coilin and coilin-Nopp140 (P=0.097), SMN-coilin and SMN-SMN (P=0.58), coilin-WRAP53 and coilin-SART3 (P=0.352). (b) Normalized FRET ratio change at 1 s stress. After stress was applied, normalized FRET ratios increased for coilin-coilin (n=41), coilin-SmE (n=9), coilin-Nopp140 (n=9), WRAP53-WRAP53 (n=8), coilin-WRAP53 (n=23), coilin-SART3 (n=11), SMN-WRAP53 (n=15), SMN-coilin (n=13), and SMN-SMN (n=6), SMN-SmG (n=11) but not for SmE-SmG (n=63), SMN-SART3 (n=73) and FBL-coilin (n=41). No significant difference was observed between coilin-coilin and coilin-Nopp140, WRAP53-WRAP53 and coilin-WRAP53, coilin-WRAP53 and SMN-WRAP53, SMN-coilin and SMN-SMN, coilin-coilin and SMN-coilin. (c) Average phase lags of SART3 (n=28), SmG (n=24), SmE (n=18), SMN (n=13), WRAP53 (n=43), coilin (n=13) and Nopp140 (n=9). The differences between these average phase lags are not significant (P>0.05) because of variations among different cells. The paired comparison between two proteins within the same CB is statistically different. (d) An oscillatory load of 0.3 Hz is applied at the cell apical surface and the phase lag between the force applied (bead displacement) and protein displacements are compared. Phase lag of YFP labelled proteins were subtracted by the phase lag of CFP-labelled proteins in the same CB, except for CFP-coilin and YFP-SMN pair, which was done in the reverse order to show the absolute value of the phase-lag difference; paired comparison was used to determine the statistical significance between each protein pair. Number of CBs for CFP-YFP pair of SmE-SmG is 20; coilin-coilin is 13; coilin-SmE is 17; coilin-Nopp140 is 11; coilin-WRAP53 is 34; coilin-SART3 is 26; SMN-WRAP53 is 24; SMN-coilin is 44; coilin-SMN is 16; SMN-SMN is 13; SMN-SmG is 24; SMN-SART3 is 10. Mean±s.e.m. data are pooled from at least 3 independent experiments (*,P<0.05; **,P<0.01).P-values were obtained using the two-tailed Student'st-test. Figure 3: Different protein complexes in the CB have distinct association characteristics. ( a ) Baseline emission ratios of SmE-SmG ( n =85), coilin-coilin ( n =56), coilin-SmE ( n =134), coilin-Nopp140 ( n =64), WRAP53-WRAP53 ( n =99), coilin-WRAP53 ( n =140), coilin-SART3 ( n =138), SMN-WRAP53 ( n =64), SMN-coilin ( n =53), SMN-SMN ( n =48), SMN-SmG ( n =100), SMN-SART3 ( n =73) and Fibrillarin (FBL)-coilin ( n =32) before stress application. No significant difference was observed between coilin-coilin and coilin-Nopp140 ( P =0.097), SMN-coilin and SMN-SMN ( P =0.58), coilin-WRAP53 and coilin-SART3 ( P =0.352). ( b ) Normalized FRET ratio change at 1 s stress. After stress was applied, normalized FRET ratios increased for coilin-coilin ( n =41), coilin-SmE ( n =9), coilin-Nopp140 ( n =9), WRAP53-WRAP53 ( n =8), coilin-WRAP53 ( n =23), coilin-SART3 ( n =11), SMN-WRAP53 ( n =15), SMN-coilin ( n =13), and SMN-SMN ( n =6), SMN-SmG ( n =11) but not for SmE-SmG ( n =63), SMN-SART3 ( n =73) and FBL-coilin ( n =41). No significant difference was observed between coilin-coilin and coilin-Nopp140, WRAP53-WRAP53 and coilin-WRAP53, coilin-WRAP53 and SMN-WRAP53, SMN-coilin and SMN-SMN, coilin-coilin and SMN-coilin. ( c ) Average phase lags of SART3 ( n =28), SmG ( n =24), SmE ( n =18), SMN ( n =13), WRAP53 ( n =43), coilin ( n =13) and Nopp140 ( n =9). The differences between these average phase lags are not significant ( P >0.05) because of variations among different cells. The paired comparison between two proteins within the same CB is statistically different. ( d ) An oscillatory load of 0.3 Hz is applied at the cell apical surface and the phase lag between the force applied (bead displacement) and protein displacements are compared. Phase lag of YFP labelled proteins were subtracted by the phase lag of CFP-labelled proteins in the same CB, except for CFP-coilin and YFP-SMN pair, which was done in the reverse order to show the absolute value of the phase-lag difference; paired comparison was used to determine the statistical significance between each protein pair. Number of CBs for CFP-YFP pair of SmE-SmG is 20; coilin-coilin is 13; coilin-SmE is 17; coilin-Nopp140 is 11; coilin-WRAP53 is 34; coilin-SART3 is 26; SMN-WRAP53 is 24; SMN-coilin is 44; coilin-SMN is 16; SMN-SMN is 13; SMN-SmG is 24; SMN-SART3 is 10. Mean±s.e.m. data are pooled from at least 3 independent experiments (*, P <0.05; **, P <0.01). P -values were obtained using the two-tailed Student's t -test. Full size image Dissipative behaviours of protein complexes in the Cajal body In a time-dependent force-deformation response, a phase lag (or a time delay), between the applied cyclic stress at the cell surface and the displacement of a nuclear protein, is a measure of the rheological properties of the material. Any viscoelastic linkage has a phase lag of between 0° and 90°. For multiple linkages of different proteins in a complex protein aggregate that is tethered in a nucleoplasmic matrix, the phase lags would indicate how viscous these interactions are. Under an oscillatory stress of 0.3 Hz, the phase lag of coilin to the magnetic bead displacement (a measure of cytoplasmic strain, which, in turn, was ~5° lagged behind the applied force; see Fig. 1b ) was ~33°, 4° more than that of SMN (~29°) inside the same CB ( Fig. 3c ). The fact that coilin was always lagged 4° behind SMN, irrespective of which fluorescent probe (CFP or YFP) was attached to coilin ( Fig. 3d ), suggests that these phase lags were not biased by the attached fluorescent probes. The phase-lag differences between CFP-coilin and YFP-coilin or CFP-SMN and YFP-SMN were almost 0° ( Fig. 3d ), suggesting that the 4°-phase difference did not originate from CFPs or YFPs themselves. The 4°-phase difference suggests that the SMN-coilin interactions are viscoelastic and dissipative. The phase-lag differences between SmE and SmG, between coilin and Nopp140, between coilin and SmE were all <2°, suggesting that the dissipative elements (where the input mechanical energy is dissipated into heat) between them were not as significant. Coilin-WRAP53, coilin-SART3, SMN-WRAP53, SMN-SmG and SMN-SART3 pairs have significant phase-lag differences between each protein pair (~2–3°, corresponding to a time delay of 20–30 ms (3° times 3,200 ms divided by 360° equals 26.7 ms; one cycle is 3,200 ms at a loading frequency of 0.3125 Hz)), indicating that force is dissipated when transmitted from one protein to the other. Interestingly, viscous responses were also evident when a sudden stress (a step function) was applied to the cell surface. The FRET curves exhibited creep responses showing local 'material deformation' (two proteins pulled apart): slow responses (creep time, defined as time to reach peak FRET change, ~700–1,350 ms) indicate a predominantly viscous behaviour ( Fig. 4a–d ); in contrast, fast responses (creep time ~300 ms, confirmed by sampling at a time resolution of ~150 ms in Fig. 4e ) are likely to be associated with more elastic local nanoenvironment ( Fig. 4f–k ). 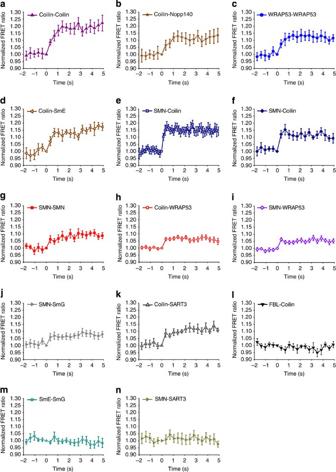Figure 4: Normalized FRET of different Cajal body protein pairs as a function of stress application duration. A step load was applied at time zero and all FRET ratios were normalized to that time point. Average data are shown for slow creep responses (creep time>700 ms) of FRET changes of coilin-coilin (a) (n=41), coilin-Nopp140 (b) (n=9), WRAP53-WRAP53 (c) (n=8), coilin-SmE (d) (n=9) and for fast creep responses (creep time <300 ms) for SMN-coilin (e) (n=10) and (f) (n=13), SMN-SMN (g) (n=6), coilin-WRAP53 (h) (n=23), SMN-WRAP53 (i) (n=15), SMN-SmG (j) (n=11), coilin-SART3 (k) (n=11). No FRET changes were observed for FBL-coilin (l) (n=41), SmE-SmG (m) (n=63), and SMN-SART3 (n) (n=73). Mean±s.e.m. data are pooled from at least three independent experiments. Figure 4: Normalized FRET of different Cajal body protein pairs as a function of stress application duration. A step load was applied at time zero and all FRET ratios were normalized to that time point. Average data are shown for slow creep responses (creep time>700 ms) of FRET changes of coilin-coilin ( a ) ( n =41), coilin-Nopp140 ( b ) ( n =9), WRAP53-WRAP53 ( c ) ( n =8), coilin-SmE ( d ) ( n =9) and for fast creep responses (creep time <300 ms) for SMN-coilin ( e ) ( n =10) and ( f ) ( n =13), SMN-SMN ( g ) ( n =6), coilin-WRAP53 ( h ) ( n =23), SMN-WRAP53 ( i ) ( n =15), SMN-SmG ( j ) ( n =11), coilin-SART3 ( k ) ( n =11). No FRET changes were observed for FBL-coilin ( l ) ( n =41), SmE-SmG ( m ) ( n =63), and SMN-SART3 ( n ) ( n =73). Mean±s.e.m. data are pooled from at least three independent experiments. Full size image Taking together the FRET changes in an intact cell and in a cell where specific components of the cytoskeleton and of the nuclear skeleton are disrupted or knocked out, we propose a working model of the force response for the protein complex in the CB ( Fig. 5 ): the protein complex is stressed via the pathway of integrin-mediated focal adhesion to F-actin, to LINC, to nuclear lamina, to a putative nucleoplasmic element (likely chromatin and/or an actin-dependent filamentous network [32] ), and then to the CB. Interestingly, at a higher loading frequency of 0.83 Hz, coilin still phase-lagged SMN by ~4°, although the magnitudes of phase lags of both proteins decreased by ~4° (to ~29° for coilin and ~25° for SMN) ( Fig. 6a ). These frequency-dependent data suggest that a more dynamic force resulted in a more elastic cytoskeleton and/or nucleoskeleton (lower phase lags or less dissipative energy). 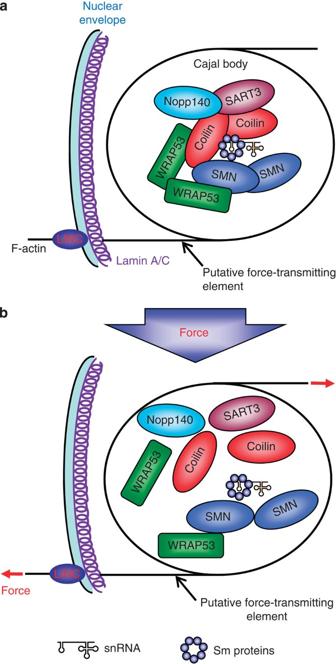Figure 5: A working model of force propagation to the Cajal body. Cajal body interactome under normal physiologic conditions (a) and under an external mechanical stress at the cell surface (b). Two major multi protein–RNA complexes in the Cajal body are characterized by coilin-mediated associations and SMN-mediated associations. We propose a working model that an incoming force transmits into the nucleus via tensed F-actin to LINC, across the nuclear envelope to nuclear lamina, then to a putative nuclear force transmitting element (likely chromatin and/or an actin-dependent nuclear filamentous network32), from there to the CB to dissociate the protein complexes. LINC, linker of nucleoskeleton to cytoskeleton; snRNA, small nuclear RNA. Figure 5: A working model of force propagation to the Cajal body. Cajal body interactome under normal physiologic conditions ( a ) and under an external mechanical stress at the cell surface ( b ). Two major multi protein–RNA complexes in the Cajal body are characterized by coilin-mediated associations and SMN-mediated associations. We propose a working model that an incoming force transmits into the nucleus via tensed F-actin to LINC, across the nuclear envelope to nuclear lamina, then to a putative nuclear force transmitting element (likely chromatin and/or an actin-dependent nuclear filamentous network [32] ), from there to the CB to dissociate the protein complexes. LINC, linker of nucleoskeleton to cytoskeleton; snRNA, small nuclear RNA. 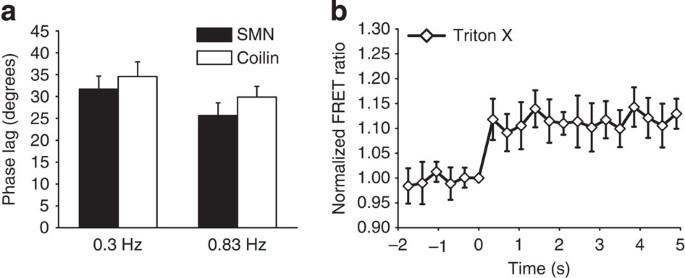Figure 6: Cajal body protein phase lags are loading-frequency dependent, and their dissociation does not depend on opening of ion channels. (a) At 0.83 Hz (n=20 CBs), phase lags between coilin or SMN and the bead displacement decreased by 4° when compared with loading at 0.3 Hz (n=44 CBs from different cells). (b) After a magnetic bead was bound, the cell was treated with 0.1% Triton X for 3.5 min to remove the plasma membrane. On stress application, a change in FRET ratio was observed.n=3 cells. Mean±s.e.m. data are pooled from three independent experiments. Full size image Figure 6: Cajal body protein phase lags are loading-frequency dependent, and their dissociation does not depend on opening of ion channels. ( a ) At 0.83 Hz ( n =20 CBs), phase lags between coilin or SMN and the bead displacement decreased by 4° when compared with loading at 0.3 Hz ( n =44 CBs from different cells). ( b ) After a magnetic bead was bound, the cell was treated with 0.1% Triton X for 3.5 min to remove the plasma membrane. On stress application, a change in FRET ratio was observed. n =3 cells. Mean±s.e.m. data are pooled from three independent experiments. Full size image In this study, we have shown that a local dynamic surface force can directly alter protein–protein associations in the CB in the nucleus of a living cell without intermediate biochemical cascades. These results provide experimental evidence supporting the proposed model of direct force propagation and transduction from ECM to the nucleus [3] . Our findings show that a local force transferred via integrins is propagated in the cytoplasm along the tensed actin cytoskeleton to the nuclear envelope, and across the nuclear envelope to the nuclear lamina, and from the nuclear lamina to a putative nuclear stress-propagating element, which might be chromatin and/or a filamentous structure, and from there to essential CB component SMN, and then to coilin, a structural element of the CB. Our recent findings on the essential roles of myosin-II-mediated tension and intact actin bundles in cytoskeletal force transmission are consistent with our earlier findings on long-distance force transmission and transduction [24] , [33] , [34] . However, previous reports show that direct activation of cytoplasmic enzyme Src or Rac by force also depends on intact microtubules, whereas here, we find that dissociation of SMN from coilin in the CB does not depend on microtubules, suggesting a difference in force transduction pathway in activation of molecules between the nucleus and the cytoplasm. It is known that the nuclear stiffness of a differentiated cell is ~5 to 10-fold higher than that of the cytoplasm [8] , [13] . One might infer that it would be difficult to displace closely interacting molecules inside the nucleus. However, our present study demonstrates that protein components in the CB can be displaced significantly by a local force of physiological magnitudes. These data suggest that a force might be focussed at the cytoskeletal-nuclear coupling on the nuclear envelope such that efficient stresses are transmitted (likely via chromatin and/or the putative nucleoplasmic filaments [32] ) to the CBs. It has been documented that Lamin A/C, expressed abundantly in differentiated cells, is an elastic scaffold to provide structural support to the nuclear envelope and nuclear stiffness [10] , [11] , [12] , [13] , [35] . One might think that knocking out Lamin A/C would soften the nucleus and make it easier to deform the nucleoplasmic proteins. In contrast, our data show that cells lacking Lamin A/C fail to transmit surface forces to the CB to dissociate coilin from SMN. These data imply that the nuclear lamina also functions as necessary force-transmitting filaments to molecules inside the nucleoplasm, supported by the data of significant Lamin A deformation, in response to the cell surface force, thus extending recent findings that the LINC complex has important roles in transmitting forces to different parts of the cytoplasm [36] , [37] . Although F-actin, intermediate filaments, or microtubules are all physically associated with the nuclear envelope via LINC or emerin [12] , our findings that plectin and microtubules do not have a significant role in force-induced dissociation of CB proteins suggest that forces are propagated into the nucleus and the CB mostly via F-actin-LINC pathway. In a physiological environment, the ECM is a flexible polymer network that mediates external forces into the living cell and ECM stiffness is known to have profound impacts on many cellular functions [26] . Our current results, showing that protein complexes in the CB dissociate in response to force only when substrate rigidity is approximately equal to or greater than the maximum cell stiffness, are consistent with previous reports but extend the role of substrate rigidity to force-induced protein–protein dissociations in the nucleus. However, whether these force-induced changes are physiologically relevant or not needs to be determined in the future in a living tissue under a normal physiological environment. It is known that mechanical forces can lead to conformational changes or unfolding of cytosplasmic proteins such as spectrin [4] , talin [5] and vinculin [38] . It is possible that, in this study, the CB components such as coilin and SMN are also partially unfolded by force. However, protein unfolding alone cannot explain the results of highly elevated MSDs in coilin but not in SMN after force application. Therefore, there must be significant dissociation or physical separation of coilin from SMN such that the two proteins are constrained by different local microenvironments after force application. In addition, the magnitudes of stress-induced displacements for coilin and SMN are too large to be accounted for by protein unfolding alone. Our findings on the phase-lag differences in different protein complexes have demonstrated for the first time viscoelastic interactions for multiple CB-interacting proteins. What might be the physiological relevance of our findings in understanding the CB structure and function? Our FRET data during force application suggest that we have identified two major multi-protein–RNA complexes in the CB. The first complex is characterized by protein associations with high affinity mediated by coilin and its self-interacting ability. The second complex is mediated by the SMN protein and its self-oligomerizing activity with low-affinity associations. Interestingly, the critical interaction for the CB integrity between coilin and SMN is not very strong, which may explain the separation of coilin-containing CB residual body from SMN-containing gem when coilin-SMN interaction is impaired [16] . It appears that WRAP53, which likely recruits the SMN protein complex to CB and mediates the interactions between SMN and coilin [27] , has a stronger affinity to coilin than to SMN. This suggests that WRAP53 is being stabilized by coilin in the CB. Because coilin mediates strong associations with its interacting partners, spliceosomal snRNPs, Nopp140, SART3, not surprisingly, these coilin interactions are more significantly affected under mechanical stress than SMN protein-mediated ones. Thus, our results provide the first in-depth in vivo readout of the major CB structural-functional interactome under normal and stress conditions. A recent view on the function of CBs suggests that the CB acts as a depot for final modifications of spliceosomal snRNPs. These are delivered to CBs by the SMN protein complex from the cytoplasm, before they function in pre-mRNA splicing in the nucleoplasm. SMN is hyperphosphorylated in the cytoplasm and able to recruit proteins to the SMN protein complex in the cytoplasm. Then, WRAP53 mediates the import of the SMN protein complex with snRNPs to CBs [35] which is recruited to CBs by hypophosphorylated coilin [39] . Importantly, in the following step snRNPs are exchanged between the SMN complex and coilin in CBs. Coilin is hyperphosphorylated on its carboxy terminus, which disrupts its interaction with SMN, promoting the release of SMN from the CB and enhancing coilin-snRNP interaction. Thus, snRNPs are transferred from SMN to coilin and become available for further modifications in CBs. As a consequence, coilin is dephosphorylated, possibly by phosphatase PPM1G, which facilitates the release of snRNPs for their functions in pre-mRNA splicing [28] . Can the results on dissociation of nuclear protein complexes be explained by indirect steps such as opening of ion channels at the plasma membrane? It has been shown previously that calcium influx and propagation in the cytoplasm, after a local stress, takes several seconds for calcium to reach a remote site of 10–20 μm away [40] , whereas we found dissociation of SMN from coilin within 0.35 s at a distance of 10–20 μm. Therefore, it would be difficult to explain our findings by calcium influx following ion channel opening. Importantly, the stress-induced FRET ratio change of SMN-coilin was still observed after short-time exposure (~3.5 min) to 0.1% Triton X to remove the plasma membrane ( Fig. 6b ), suggesting that ion channel opening may not be important in force-induced dissociation of proteins complexes in the CB. However, our current findings do not rule out the important roles of slow processes (for example, diffusion and/or translocation) induced by force in cellular remodelling and biological responses, which might be synergistic, non-synergistic, or antagonistic with those by soluble growth factors. In this study, FRET changes were also observed in mouse skin fibroblasts (besides HeLa cells) in response to force, suggesting that the force-induced dissociation of protein complexes in the nucleus may represent a generalized response from different types of differentiated cells. Interestingly, CBs that exhibit FRET changes in response to force are the ones that show spontaneous constrained-diffusion ( Fig 1h ), whereas some CBs that do not respond to force in general exhibit simple diffusion [41] , and thus may be only loosely associated with chromatin, consistent with published data that association of CBs to chromatin significantly affects their dynamics [20] . Thus, CBs are likely to have an important regulatory role in expression of specific genes with which they are physiologically associated. However, at the present time, there are no techniques available that have the capability to measure gene expression fast and specifically enough in a single cell to explain the direct force effect. In the future, it would be interesting to assess if such methods can be developed to determine whether responses of CBs to force are important in regulating expression of specific genes. Our findings that force propagation from cell surface receptors integrins to SMN-coilin in the nucleus is blocked in Lamin A/C−/− cells may have implications in the premature ageing disease Hutchinson–Gilford Progeria Syndrome [42] . Recent findings have also revealed the importance of mechanical forces in ECM-integrin-cytoskeleton-myosin-II-dependent cancer progression [43] , [44] , [45] . As CBs are predominantly present in transformed or aneuploid cancer cells, it is conceivable that mechanical forces on cell surface might have a direct impact on cell transformation via altering the dynamics of components of nuclear bodies. In summary, we have demonstrated that dynamic force can induce direct structural changes of essential components of a major nuclear body, which may represent a unique mechanism of mechanotransduction that impacts on gene expression and genome maintenance. Cell culture and transfection HeLa cells, LMNA-knockout mouse embryonic fibroblast cells, and plectin knockout mouse skin fibroblasts were cultured and maintained in DMEM (Sigma) supplemented with 10% FBS (HyClone), 100 U ml −1 penicillin, 100 μg ml −1 streptomycin and 2 mM L -Glutamine at 37 °C in 5% CO 2 . For live cells imaging, cells were plated on glass bottom dishes coated with type I collagen (40 μg ml −1 ), overnight. Each fluorescence protein plasmid of interest was transfected at 1 μg per 35 mm glass bottom dish using Lipofectamine 2000,20 h before experiment, following protocols provided by the manufacturer (Invitrogen). The plasmids CFP-SMN [14] , [46] , YFP-SMN [14] , [46] , CFP-coilin [47] , YFP-Coilin [47] , fibrillarin-YFP [48] constructs are described as referenced. YFP-Nopp140, CFP-WRAP53, YFP-WRAP53, YFP-SART3, CFP-SmE, YFP-SmE, CFP-SmG and YFP-SmG were subcloned into either pECFP-C1 or pEYFP-C1 expression vectors as indicated. mCherry-Lamin A plasmid was a gift from Dr. P. Kalab. The cell culture media was then changed 6 h after transfection to serum-deprived-media. Magnetic twisting cytometry and cell stiffness The optical magnetic twisting cytometry method [49] , [50] was used to exert mechanical stress on the living HeLa cells. Arg-Gly-Asp (RGD)-coated ferromagnetic beads (Fe 3 O 4 , ~4 μm in diameter) were added to the cells and then incubated for 10 min to allow for integrin clustering and formation of focal adhesions surrounding the bead. The beads were magnetized in the horizontal direction by a strong magnetic pulse (1,000 G) for a brief period (<100 μs). During imaging, cells were maintained in CO 2 -independent medium without serum (Invitrogen) at 37 °C. Cell Young's modulus in Pa was estimated by quantifying the embedded area of the magnetic bead and using the cell stiffness data (in Pa per nm) [51] . Fluorescent beads (0.2 μm in diameter) were embedded in the polyacrylamide gel substrate, and their positions were recorded by fluorescence microscopy. The displacement field induced by each individual cell's tractional forces was determined by comparing the fluorescent bead positions before and after trypsinization (cell-free and thus force-free). The RMS (root-mean-square) traction was calculated from the displacement field with known substrate stiffness [52] . Cell tractions were quantified after the cells were plated on various stiffnesses (0.6, 2 and 8 kP, corresponding to 0.06% bisacrylamide and 3% acrylamide, 0.05% bisacrylamide and 5% acrylamide, 0.3% bisacrylamide and 5% acrylamide, respectively) of collagen-1-coated polyacrylamide gels [52] . For FRET imaging, the magnetic twisting field (0, 1.8, 3.5, 8.8, 14, 17.5, or 24.5 Pa) was applied as a step function (a constant magnetic field) to the magnetic beads that are bound to the surface of the cells. A Leica inverted microscope was integrated with a magnetic twisting device and a Dual-View system (Optical Insights) to simultaneously acquire both CFP and YFP emission images in response to stress. CFP/YFP Dual EX/EM (FRET) (OI-04-SEX2) has the following filter sets: CFP: excitation, S430/25, emission S470/30; YFP: excitation, S500/20, emission S535/30. The emission filter set uses a 515-nm dichroic mirror to split the two emission images. For FRET imaging, we excited at CFP wavelength and measured the emission of both CFP and YFP simultaneously on the same screen using a CCD camera (Hamamatsu C4742-95-12ERG) and a 63×1.32 N.A. oil-immersion objective. Exposure time was 290 ms or 150 ms. For CB dynamics imaging, an oscillatory magnetic field (24.5 Pa at 0.3 or 0.83 Hz) was applied. CFP-SMN and YFP-Coilin images before, during and after mechanical loading were captured at every 0.32 or 0.09 s interval over a period of ~15 s, respectively. Bright-field images of the cell and the magnetic bead during oscillatory load were also obtained for bead displacement analysis. To minimize photobleaching, the cells were treated with 0.5 mM Trolox (6-Hydroxy-2,5,7,8-tetramethylchroman-2-carboxylic acid; Sigma) 18 h (ref. 53 ) before imaging and illuminated with 12% light intensity by using a 120-W Hg lamp (Leica). Statistical analysis A two-tailed Student's t -test was used for all statistics. Technical issues related to FRET analyses Are there potential spontaneous movement artefacts caused by moving structures inside the nucleus? It is known that the largest speed of Cajal body movement can reach ~0.9 μm min −1 (15 nm s −1 ) [41] , which may account for the observed spontaneous movements of the CBs in our study. However, we have observed that, in spontaneous movements of CBs before force application, there is no separation of coilin from SMN, that is, both proteins move at the same rate, and thus there is no FRET change of the protein complex. More importantly, the anti-correlation behaviour between CFP-SMN (increase in emission) and YFP-coilin (decrease in emission) and differential displacements between SMN and coilin in response to force provide a strong evidence that the ratio changes are force-induced FRET changes and not movement artefacts. In addition, we excited at CFP wavelength and simultaneously measured emissions from both CFP and YFP without any time delay. The CFP-SMN transfection (without transfection of YFP-coilin) and excitation yielded only a minimal leak through the YFP channel emission. Therefore, the CFP/YFP ratio change is a measure of FRET change that is due to association or dissociation of one protein from the other by force. As we compared this FRET change in the absence and the presence of applied stress, any bleaching and/or spontaneous FRET changes are accounted for or normalized. Image analysis A customized Matlab (Mathworks) program was used to obtain CFP/YFP emission ratio and CB displacement map. For CFP/YFP emission ratio analysis, CFP and YFP images at each time point were first background-substracted, and aligned pixel-by-pixel by maximizing the normalized cross-correlation coefficient of CFP and YFP images. YFP image was then thresholded to generate a binary mask so that the pixel value inside the fluorescent particle was set to 1, and that outside the fluorescent particle was set to 0. Aligned CFP/YFP emission ratios were displayed as a linear pseudocolour. To obtain the displacement field of Coilin and SMN, CFP and YFP images were divided into small arrays of 11×11 pixels that overlap by 5 pixels. The corresponding arrays at the same location between two adjacent images taken at different phases during the twisting cycle were compared in the Fourier domain. This sensitive method can detect displacements of the fluorescent particles to the resolution of 4–5 nm (ref. 54 ). For Cajal body dynamics analysis, a custom Matlab program was developed to convert the fluorescent image into black and white. The centroid coordinates of each fluorescence particle obtained from the binary image were used to calculate the MSD of coilin and SMN. The MSD before, during, and after mechanical loading were calculated based on equation (1) where r ( t ) is the fluorescence particle position and Δ t is the time step (0.32 s in our case). The same procedure is performed on bright-field images to obtain the magnetic bead MSD . How to cite this article: Poh, Y.-C. et al . Dynamic force-induced direct dissociation of protein complexes in a nuclear body in living cells. Nat. Commun. 3:866 doi: 10.1038/ncomms1873 (2012).